Few-layer molybdenum disulfide transistors and circuits for high-speed flexible electronics Two-dimensional layered materials, such as molybdenum disulfide, are emerging as an exciting material system for future electronics due to their unique electronic properties and atomically thin geometry. Here we report a systematic investigation of MoS 2 transistors with optimized contact and device geometry, to achieve self-aligned devices with performance including an intrinsic gain over 30, an intrinsic cut-off frequency f T up to 42 GHz and a maximum oscillation frequency f MAX up to 50 GHz, exceeding the reported values for MoS 2 transistors to date ( f T ~0.9 GHz, f MAX ~1 GHz). Our results show that logic inverters or radio frequency amplifiers can be formed by integrating multiple MoS 2 transistors on quartz or flexible substrates with voltage gain in the gigahertz regime. This study demonstrates the potential of two-dimensional layered semiconductors for high-speed flexible electronics. Two-dimensional layered materials (2DLMs), such as graphene or molybdenum disulfide (MoS 2 ), are emerging as an exciting material system for future electronics due to their unique electronic properties and atomically thin geometry [1] , [2] , [3] , [4] , [5] , [6] , [7] , [8] . Graphene has been explored for ultrahigh-speed transistors with the intrinsic cut-off frequency exceeding 400 GHz [9] , but typically with insufficient current on–off ratio and little voltage gain due to its zero band gap semimetal nature. Alternatively, the semiconducting MoS 2 has recently drawn considerable interest for overcoming these disadvantages of graphene to enable atomically thin transistors with high on–off ratio and intrinsic voltage gain [10] , [11] , [12] , [13] , [14] , [15] , [16] , [17] . A single layer of MoS 2 consists of a layer of Mo atoms sandwiched between two layers of S atoms. As a 2D material, it shares many interesting characteristics of the well-known graphene such as atomically thin thickness, excellent electronic properties, high mechanical flexibility and partial optical transparency [1] , [3] . With a direct band gap of 1.8 eV (refs 7 , 8 ), it overcomes the key shortcomings of graphene for electronic applications—the lack of band gap and unsatisfying current saturation [18] . 2D electronics based on single- or few-layer MoS 2 represents the ultimate limit of thickness for pushing the limits of the Moore’s law. With a larger band gap than silicon and atomically thin geometry, MoS 2 is also advantageous for suppressing the source-to-drain tunnelling current in ultra-short transistors at the scaling limit and offers superior immunity to short-channel effects [19] . Moreover, MoS 2 and other transition metal dichalcogenide (TMD) materials are attractive as an alternative material for low-cost flexible electronics that is currently dominated by amorphous silicon, organic semiconductors or low-temperature-processed oxide semiconductors with carrier mobilities typically below 10 cm 2 V −1 s −1 [20] , [21] , [22] , [23] , [24] . Finally, with a 2D geometry, the atomically thin TMD may also offer excellent scalability for large scale integration, much like conventional planar electronics. A key step to realize the electronic application using 2DLMs is the demonstration of integrated circuits functioning in the gigahertz frequency regime. However, the MoS 2 circuits reported to date can only function in a few megahertz or even lower frequency regime [10] , [12] , [13] , [25] . The difficulties in integrating high-quality dielectrics and performing subtractive lithography on atomically thin materials have prevented achieving 2DLMs transistors with optimized device geometry and performance [26] , [27] , [28] , [29] . It is a well-recognized challenge to integrate dielectrics with graphene because of the intrinsic incompatibility of graphene with typical oxide dielectrics or their deposition processes [26] . Despite several attempts to date [3] , [27] , [28] , [29] , the integration of high-quality high- k dielectrics on TMDs such as MoS 2 is facing a similar challenge [27] , [29] . Furthermore, another significant challenge to achieve high-performance devices based on these atomically thin materials is their intrinsic incompatibility with the conventional subtractive lithography processes (for example, various plasma etching) that can severely damage the atomic structure and degrade the electronic properties. Here we report the state-of-the-art MoS 2 transistors by using an additive lithography approach to integrate few-layer MoS 2 with transferred gate stacks [9] . The transfer-gate strategy can allow for a damage-free process to integrate MoS 2 with high-quality dielectrics and self-aligned gate to achieve MoS 2 transistors with optimized device geometry and performance, including excellent on–off ratio, current saturation and an intrinsic gain over 30. On-chip microwave measurements demonstrate a highest intrinsic cut-off frequency f T of 42 GHz and a maximum oscillation frequency f MAX of 50 GHz. Furthermore, we have, for the first time, demonstrated the integration of multiple MoS 2 transistors on quartz and flexible substrates to form a logic inverter or radio frequency (RF) amplifier with voltage gain up to the gigahertz regime. Device fabrication Our initial studies are based on mechanically exfoliated few-layer MoS 2 flakes on Si/SiO 2 (300 nm) substrate, which were characterized by using optical microscope, atomic force microscopy and Raman spectroscopy ( Supplementary Fig. 1 ) [2] , [3] , [30] . The same process should be applicable to the large-area MoS 2 or other 2DLMs grown by chemical vapour deposition approach. The gate stacks—metal bars wrapped in dielectrics—were first patterned on a sacrificial substrate, and then transferred onto the few-layer MoS 2 (see Methods and Supplementary Fig. 2 for further details) [9] . Following electron (E)-beam lithography, a metallization (titanium (50 nm)/gold (50 nm)) process was used to define the external source, drain and gate electrodes. A thin layer of Ni/Au (5 nm/10 nm) was then deposited to form the self-aligned source and drain electrodes with minimized access resistance or parasitic capacitance [9] , [31] ( Fig. 1a ). 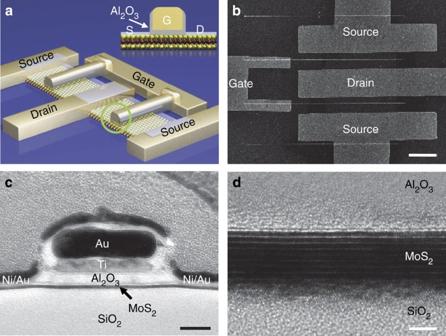Figure 1: Schematic illustration and characterization of the self-aligned MoS2transistors. (a) A schematic illustration of a dual-channel self-aligned MoS2FETs with transferred gate stacks, and the inset shows the schematic cross-section of the self-aligned device. (b) The SEM image of MoS2FETs with transferred gate stacks. Scale bar, 5 μm. (c) The cross-sectional TEM image of a typical self-aligned device. Scale bar, 50 nm. (d) HRTEM image of the interface between MoS2and the transferred gate stack. Scale bar, 3 nm. Figure 1b shows a scanning electron microscopy (SEM) image of the top view of top-gated dual-channel self-aligned MoS 2 field-effect transistors (FETs). The cross-sectional transmission electron microscope (TEM) image shows that the self-aligned source and drain electrodes are well separated and precisely positioned next to the gate spacer dielectrics ( Fig. 1c ). High-resolution TEM image shows an eight-layer MoS 2 flake with clear interface between the transferred gate stack and MoS 2 surface ( Fig. 1d ). Since phonon scattering and roughness scattering can severely degrade the mobilities in atomically thin 2D materials, a high-quality high- k dielectric with clean interface can screen the scattering and enhance the mobility of MoS 2 devices [3] . Figure 1: Schematic illustration and characterization of the self-aligned MoS 2 transistors. ( a ) A schematic illustration of a dual-channel self-aligned MoS 2 FETs with transferred gate stacks, and the inset shows the schematic cross-section of the self-aligned device. ( b ) The SEM image of MoS 2 FETs with transferred gate stacks. Scale bar, 5 μm. ( c ) The cross-sectional TEM image of a typical self-aligned device. Scale bar, 50 nm. ( d ) HRTEM image of the interface between MoS 2 and the transferred gate stack. Scale bar, 3 nm. Full size image d.c. performance The basic electronic properties of MoS 2 FETs were first probed using standard back-gate devices on Si/SiO 2 substrate (without top-gate). The transfer characteristics are determined by measuring the drain-source current I ds as a function of the back-gate voltage V BG at a fixed drain voltage V ds ( Fig. 2a ). The field-effect mobility of the device can be derived using μ =(d I ds /d V BG )·( L /( W · C 0 · V ds )), where channel length L =1 μm, channel width W =4 μm and back-gate capacitance C 0 = ε 0 ε r / d =11.5 nF cm −2 . A field-effect mobility of μ =170 cm 2 (V s) −1 at a drain voltage of V ds =0.5 V can be derived from the transconductance curve shown in left axis of Fig. 2a . This value is comparable to the best mobility values reported for MoS 2 FETs to date [1] , [3] , [5] . 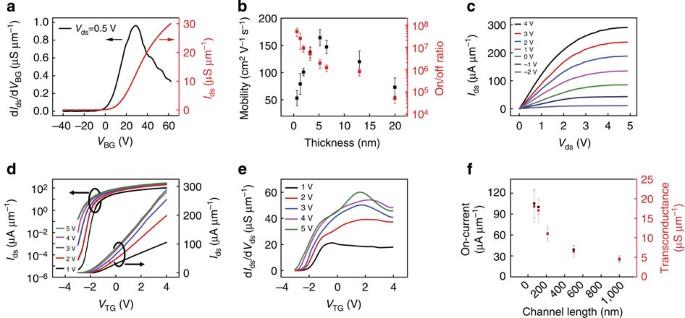Figure 2: Room-temperature d.c. characterizations of the self-aligned MoS2transistors. (a) TheIds–VBGtransfer characteristics and the corresponding transconductance of the device at 0.5 V bias voltage for the 1 μm channel length back-gated MoS2transistor. (b) The distribution of MoS2transistor mobility and on–off ratio in back-gate configuration versus thickness of MoS2. (c)Ids–Vdsoutput characteristics at various gate voltages (VTGfrom −2 to 4 V) for a 116 nm channel length top-gated MoS2transistor with self-aligned source and drain electrodes. (d) TheIds–VTGtransfer characteristics at different bias voltage for a 116 nm channel length top-gate configuration MoS2transistor with self-aligned source and drain electrodes (Vds=1, 2, 3, 4 and 5 V). (e) The corresponding transconductance of the MoS2transistor shown indat different bias voltage. (f) The distribution of on-state current and transconductance atVsd=1 V versus channel length in top-gated MoS2transistors with self-aligned source and drain electrodes. Figure 2: Room-temperature d.c. characterizations of the self-aligned MoS 2 transistors. ( a ) The I ds – V BG transfer characteristics and the corresponding transconductance of the device at 0.5 V bias voltage for the 1 μm channel length back-gated MoS 2 transistor. ( b ) The distribution of MoS 2 transistor mobility and on–off ratio in back-gate configuration versus thickness of MoS 2 . ( c ) I ds – V ds output characteristics at various gate voltages ( V TG from −2 to 4 V) for a 116 nm channel length top-gated MoS 2 transistor with self-aligned source and drain electrodes. ( d ) The I ds – V TG transfer characteristics at different bias voltage for a 116 nm channel length top-gate configuration MoS 2 transistor with self-aligned source and drain electrodes ( V ds =1, 2, 3, 4 and 5 V). ( e ) The corresponding transconductance of the MoS 2 transistor shown in d at different bias voltage. ( f ) The distribution of on-state current and transconductance at V sd =1 V versus channel length in top-gated MoS 2 transistors with self-aligned source and drain electrodes. Full size image To evaluate the layer thickness-dependent electronic properties, we have measured more than 40 MoS 2 devices in back-gate configurations. In general, a thinner MoS 2 can usually offer a lower off-state current, but a thicker one has a larger on-state current [10] ( Supplementary Fig. 3 ). The origin of the thickness dependence of MoS 2 FET performance is a complicated issue and may be partly attributed to partial screening of electric field by the bottom layers, interlayer resistance [32] and/or Coulomb scattering effect from the substrate [33] . For even thicker MoS 2 (>20 nm), the back gate can hardly turn the channel on or off due to the increasing screening effect of the bottom layers [34] . A plot of mobility versus thickness shows that a MoS 2 with a thickness between 2 and 7 nm exhibits both the high mobility and high on–off ratio ( Fig. 2b ). Therefore, we have mainly focused on the MoS 2 flakes with a thickness between 2 and 7 nm for the fabrication of high-performance MoS 2 FETs in the following studies. To probe the performance limit of few-layer MoS 2 FETs, we have fabricated top-gated short-channel devices with self-aligned source and drain electrodes (Ni/Au) to minimize the access resistance and parasitic capacitance. The output characteristics of a 116 nm channel length self-aligned MoS 2 transistor were measured at various top-gate voltages ( Fig. 2c ). The I ds – V ds curve shows linear behaviour at low bias voltages, suggesting that the self-aligned Ni/Au thin film forms Ohmic contacts with MoS 2 (ref. 31 ). We have also performed temperature-dependent measurement and a perfect linear I ds − V ds curve is observed at 30 K, demonstrating that the MoS 2 metal contact barrier is much smaller than 2.6 meV and negligible at room temperature (see Supplementary Fig. 4 ). Significantly, a clear current saturation is observed at high source-drain bias, which is difficult to achieve in graphene transistors with such a short channel length. The drain-source conductance g ds =d I ds /d V ds is close to zero in this region of operation (see Supplementary Fig. 5 ). Current saturation is a very important parameter for achieving maximum possible operating speeds [35] . The transfer characteristics ( I ds – V TG curves) of the same device were measured at different drain bias ( Fig. 2d ). Our study shows typical n-type FET characteristics with the threshold voltage located at around −2 V. Importantly, an on/off ratio exceeding 10 7 is achieved in this device, sufficient for typical logic circuits [36] , which cannot be achieved in graphene-based devices. The subthreshold swing, defined as S =(d V TG /d(log I ds )), S =158 mV per dec can be extracted at V ds =1 V. In conventional metal–oxide–semiconductor field-effect transistors, the subthreshold swing depends on the ratio of gate capacitance to the other parasitic capacitance such as interface trap-state capacitance, and has a theoretical limit of 60 mV per dec at room temperature. A steep subthreshold swing is generally desirable for low-power operation. The transconductance, defined as g m =d I ds /d V TG , can also be derived from I ds − V TG characteristics’ curves ( Fig. 2e ). A peak scaled transconductance of 60 μS μm −1 is obtained at V ds =5 V, which represents the highest transconductance value reported for MoS 2 FETs to date [37] . The ratio of transconductance to drain-source conductance defines the intrinsic gain ( A = g m / g ds ), which is an important figure of merit representing the highest achievable gain in a single transistor [18] . With record high values of transconductance ( g m =60 μS μm −1 for V ds =5 V) and clear current saturation ( g ds <2 μS μm −1 under the same source-drain and gate bias), an intrinsic gain over 30 can be achieved in the 116 nm MoS 2 transistors ( Supplementary Fig. 5 ). This is in stark contrast to graphene transistors with similar channel length in which intrinsic gain cannot be achieved due to little current saturation in output characteristics. Such high intrinsic gain observed in the MoS 2 transistors can address the critical limit of graphene-based transistors to open up exciting potential for both digital and analogue applications with voltage gain. We have also studied the self-aligned MoS 2 transistors with variable channel lengths. The I ds – V TG transfer curves were measured from more than 30 devices with self-aligned gate lengths ranging from 68 nm to 1 μm. The distributions of on-state current and transconductance with different channel lengths were extracted from the I ds – V TG transfer curves. In general, both the on-state current and the transconductance increase with decreasing channel length ( Fig. 2f ), suggesting that the MoS 2 channel dominates the charge transport and the self-aligned Ni/Au contacts form good contacts with MoS 2 . The contact resistance of Ni/Au contact can be measured by using transfer length method ( Supplementary Fig. 6 ). An on-state contact resistance (the contact resistance when the device is switched on by a positive gate voltage) as low as 2.5 kΩ μm can be extracted in the Ni/Au contact MoS 2 device. The total resistance of a 68 nm channel length MoS 2 transistor is ~15 kΩ μm under working condition, indicating that the contact resistance does not dominate the transport property of MoS 2 device. This is different from graphene devices, in which the channel resistance (~30 Ω μm) is much smaller than the contact resistance (~200 Ω μm) [9] . RF performance The above discussions clearly demonstrate that our self-aligned devices exhibit the best d.c. performance achieved in MoS 2 FETs to date. To further evaluate the RF performance, we have conducted the on-chip microwave measurements to determine the cut-off frequency ( f T ), using an Agilent 8361A network analyzer in the range of 50 MHz–30 GHz. The MoS 2 transistors for RF measurement were fabricated on highly resistive silicon substrate (>18,000 Ω cm) to minimize the parasitic capacitance. To accurately assess the intrinsic f T value, careful de-embedding procedures were performed using the exact pad layout as ‘open’ and ‘short’ structures on the same chip (see Methods for further details) [9] , [38] , [39] , [40] , [41] , [42] . The de-embedded S parameters constitute a complete set of coefficients describing intrinsic input and output behaviour of MoS 2 transistors. The small-signal current gain | h 21 | extracted from the measured S parameters exhibits a typical 1/ f frequency dependence expected for an ideal FET ( Fig. 3a ). The linear fit yields cut-off frequencies f T =13.5, 26 and 42 GHz for the transistors under a d.c. bias of 5 V with channel lengths of 216 nm (blue triangle in Fig. 3a ), 116 nm (red circle) and 68 nm (black square), respectively. These values were further verified by using Gummel’s approach ( Fig. 3a , inset) [43] . To the best of our knowledge, the observed f T value of 42 GHz is the highest cut-off frequency obtained in all TMD-based transistors reported to date, far exceeding the best values reported previously (0.9 GHz) [44] . 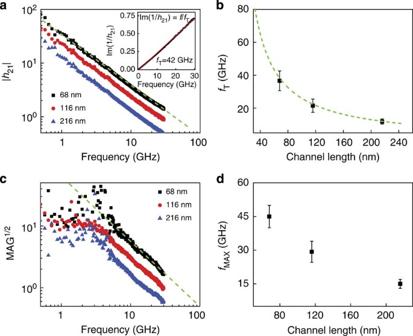Figure 3: RF performance of the self-aligned MoS2transistors. (a) Small-signal current gain |h21| versus frequency for three devices with a channel length of 216 nm (blue), 116 nm (red) and 68 nm (black) at room temperature. The cut-off frequencies are 13.5, 26 and 42 GHz at a d.c. bias of 5 V and gate bias of 2.1, 2.3 and 1.9 V, respectively. (b) PeakfTas a function of gate length from over 20 MoS2FETs. (c) Maximum available gain (MAG) versus frequency for three devices shown inawith a channel length of 216 nm (blue), 116 nm (red) and 68 nm (black) at room temperature. The maximum oscillation frequency (fMAX) are 16, 34 and 50 GHz at a d.c. bias of 5 V and gate bias of 2.1, 2.3 and 1.9 V, respectively. (d) PeakfMAXas a function of gate length from over 20 MoS2FETs. Figure 3: RF performance of the self-aligned MoS 2 transistors. ( a ) Small-signal current gain | h 21| versus frequency for three devices with a channel length of 216 nm (blue), 116 nm (red) and 68 nm (black) at room temperature. The cut-off frequencies are 13.5, 26 and 42 GHz at a d.c. bias of 5 V and gate bias of 2.1, 2.3 and 1.9 V, respectively. ( b ) Peak f T as a function of gate length from over 20 MoS 2 FETs. ( c ) Maximum available gain (MAG) versus frequency for three devices shown in a with a channel length of 216 nm (blue), 116 nm (red) and 68 nm (black) at room temperature. The maximum oscillation frequency ( f MAX ) are 16, 34 and 50 GHz at a d.c. bias of 5 V and gate bias of 2.1, 2.3 and 1.9 V, respectively. ( d ) Peak f MAX as a function of gate length from over 20 MoS 2 FETs. Full size image To further investigate the reproducibility of our approach and examine the length-scaling relationship, we have systematically examined more than 20 MoS 2 transistors of variable channel lengths ( Fig. 3b ). In general, the peak cut-off frequencies follow 1/ L dependence. A similar 1/ L dependence is usually observed in short-channel conventional Si and III–V FETs, which is mainly due to the nearly constant effective carrier velocity obtained by reaching the saturation velocity of the channel material [45] . Similarly, the 1/ L scaling trend observed in our devices is originated from carrier velocity saturation, which is different from that in graphene devices that are limited by contact resistance [9] (see Supplementary Fig. 6 ). The saturation velocity of carriers in our MoS 2 transistor can be estimated by using the equation: where L is the channel length (68 nm), τ is the carrier transit time and f T is the intrinsic cut-off frequency (42 GHz). On the basis of this relationship, we can extract the saturation velocity V sat ~1.8 × 10 6 cm s −1 , which is consistent with previous studies [46] . The operation of our MoS 2 devices in the saturation region is very important for achieving maximum possible operating speeds and stable operation of linear amplifiers [35] , [47] . We believe that the RF performance of our device can be further enhanced by further optimizing the contact resistance and/or improving gate coupling. In addition to cut-off frequency ( f T ), maximum oscillation frequency ( f MAX ), defined as the frequency at which the power gain is equal to one, is another important figure of merit defining the RF performance of a transistor. The maximum available gain was extracted from the measured S parameters ( Fig. 3c ). Importantly, f MAX of 16, 34 and 50 GHz can be achieved in MoS 2 transistors under a d.c. bias of 5 V with channel lengths of 216 nm (blue triangle), 116 nm (red circle) and 68 nm (black square), respectively. These values greatly exceed the best f MAX values reported for MoS 2 transistors to date (~1 GHz) [44] . To the best of our knowledge, this is also the highest maximum oscillation frequency obtained in any TMD-based material to date. Similar to the case of f T , f MAX possesses a monotonic behaviour when the channel length decreases ( Fig. 3d ). However, the trend of f MAX does not follow the 1/ L dependence. This can be attributed to the competing contributions from f T , gate resistance and output conductance g ds as the gate length decreases. The power gain performance of the MoS 2 devices may be further improved by improving the MoS 2 crystal quality, reducing substrate/environmental scattering, decreasing the gate resistance by using T-gate and/or improving the saturation behaviour of the MoS 2 devices through gate dielectric downscaling. We have also measured the RF performance of our devices on highly resistive silicon substrate without de-embedding procedure. A cut-off frequency ( f T ) of 1.3 GHz and a maximum oscillation frequency ( f MAX ) of 1.5 GHz are achieved for a 68 nm channel length MoS 2 transistor (see Supplementary Fig. 7 ), which is greatly lower than the de-embedded values. This large difference was commonly seen in previous studies of graphene transistors on silicon substrates [38] , [40] , and can be largely attributed to relatively large parasitic pad capacitance on silicon substrate. To further validate the de-embedding procedure, we have carefully analysed the S parameters and derived the device component values (including gate-source capacitance, gate-drain capacitance, transconductance, source resistance and drain resistance; Supplementary Table 1 ). The RF measurement-derived component values are highly consistent with those obtained from the d.c. measurements and finite element simulations ( Supplementary Fig. 8 ), confirming the validity of the RF measurements and the de-embedding procedures. Importantly, the parasitic pad capacitance can be greatly reduced by fabricating the device on insulating glass substrate, with which an extrinsic cut-off frequency of 10.2 GHz and a maximum oscillation frequency of 14.5 GHz have been achieved without de-embedding procedures (see Supplementary Fig. 7b ). RF circuits on quartz With excellent on–off current ratio, intrinsic gain, intrinsic cut-off frequency, power gain performance, as well as high extrinsic cut-off and maxim oscillation frequency on quartz substrate, the MoS 2 transistors can be used to construct the digital and analogue electronics in the gigahertz regime. To this end, we have fabricated an inverter circuit by connecting an enhancement-mode (E-mode) MoS 2 transistor with a resistor (formed by connecting the gate of a transistor directly to source electrode; Fig. 4a ). To minimize the parasitic capacitance for high-frequency measurement, the inverter circuit was fabricated on quartz substrate. An inverter circuit is a basic logic element that outputs a voltage representing the opposite logic level to its input. The quality of a logic inverter is often evaluated using its voltage transfer curve ( Fig. 4b ), which is a plot of input voltage versus output voltage. The slope of the transition region in the transfer curve defines voltage gain. Importantly, a voltage gain >10 is achieved in our MoS 2 -based inverter circuit ( Fig. 4b ). The achievement of a larger than unity gain demonstrates that the self-aligned MoS 2 devices can be used for the fabrication of integrated circuits for high-performance logic operations at room temperature. 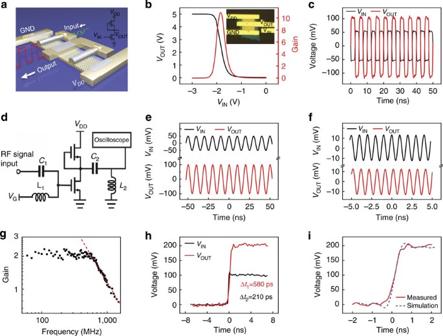Figure 4: Gigahertz logic inverter and signal amplifier based on MoS2transistors on quartz substrate. (a) Schematic illustration of an integrated logic inverter made with two MoS2transistors. (b) Output voltage (left axis) and voltage gain (right axis) of the integrated logic MoS2inverter as a function of the input voltage, highlighting a voltage gain >10. The inset shows an optical image of an integrated logic inverter on quartz substrate. (c) Input (black) and output (red) signals of the few-layer MoS2inverter under a d.c. bias of 5 V. The input signal is a 200 MHz square wave signal with amplitude of 100 mV and −1.3 V d.c. gate bias. The output signal is shifted in phase by 180° with a gain of 2 over the input signal. (d) Schematic of an integrated RF amplifier made by integrating two MoS2FETs. (e) Sinusoidal input signal (100 MHz; black) coupled with −0.5 V d.c. gate bias, and the output signal with a voltage gain of 2. (f) Sinusoidal input signal (1 GHz; black) coupled with −0.5 V d.c. gate bias, and the output signal with a voltage gain of 1.07. The d.c. bias applied on the amplifier is −6 V. (g) The frequency dependence of the small-signal voltage gain in few-layer MoS2amplifier. (h) Propagation delay of few-layer MoS2amplifier. The input signal (black) has a rise time of 210 ps and output signal (red) has a rise time of 580 ps. (i) Simulation of the propagation delay based on the frequency-dependent gain of few-layer MoS2amplifier. Figure 4: Gigahertz logic inverter and signal amplifier based on MoS 2 transistors on quartz substrate. ( a ) Schematic illustration of an integrated logic inverter made with two MoS 2 transistors. ( b ) Output voltage (left axis) and voltage gain (right axis) of the integrated logic MoS 2 inverter as a function of the input voltage, highlighting a voltage gain >10. The inset shows an optical image of an integrated logic inverter on quartz substrate. ( c ) Input (black) and output (red) signals of the few-layer MoS 2 inverter under a d.c. bias of 5 V. The input signal is a 200 MHz square wave signal with amplitude of 100 mV and −1.3 V d.c. gate bias. The output signal is shifted in phase by 180° with a gain of 2 over the input signal. ( d ) Schematic of an integrated RF amplifier made by integrating two MoS 2 FETs. ( e ) Sinusoidal input signal (100 MHz; black) coupled with −0.5 V d.c. gate bias, and the output signal with a voltage gain of 2. ( f ) Sinusoidal input signal (1 GHz; black) coupled with −0.5 V d.c. gate bias, and the output signal with a voltage gain of 1.07. The d.c. bias applied on the amplifier is −6 V. ( g ) The frequency dependence of the small-signal voltage gain in few-layer MoS 2 amplifier. ( h ) Propagation delay of few-layer MoS 2 amplifier. The input signal (black) has a rise time of 210 ps and output signal (red) has a rise time of 580 ps. ( i ) Simulation of the propagation delay based on the frequency-dependent gain of few-layer MoS 2 amplifier. Full size image Although MoS 2 transistor-based circuits have been demonstrated previously, these circuits typically operate within a few megahertz or even lower frequency regime [10] , [12] , [13] , [44] . With excellent d.c. performance and minimized parasitic capacitance on quartz substrate, our MoS 2 transistors can be readily used to construct RF circuits up to the gigahertz frequency regime. For example, with input signal of 200 MHz square wave applied to the input electrode of our MoS 2 inverter, an inverted signal with a relative voltage gain of 2 (6 dB) can be obtained at an operating frequency of 200 MHz without any noticeable delay ( Fig. 4c ). It is important to note that our inverter performance does not exclude any parasitic capacitances (such as C pg , C pd and so on) or series resistance, which highly depend on the exact circuit design. An optimized circuit design, a thinner dielectric layer or a larger bias can further improve the high-frequency performance of MoS 2 -based inverters. With much higher voltage gain than graphene transistors, the MoS 2 transistors can also be used to construct RF amplifiers ( Fig. 4d ). The amplifier is obtained by integrating two transistors in series, where the upper one acts as a ‘load’ and the lower one acts as an active ‘switch’. The gate of ‘switch’ transistor acts as input, whereas the gate of the ‘load’ transistor is connected to the central lead and acts as the output. To maximize the performance of the amplifier, the power supply of the amplifier is set at −6 V. A small sinusoidal signal V IN is superimposed on the d.c. bias V g via a bias-T. The output signal V OUT is connected to and monitored by an oscilloscope via a d.c. blocker. When a 100 MHz sinusoidal wave with amplitude of 100 mV peak-to-peak voltage was applied on the input electrode, a sinusoidal wave with larger amplitude can be observed in the output signal ( Fig. 4e ). Comparing the output signal versus the input signal, a relative voltage gain of 2 can be achieved. Furthermore, the amplifier exhibited a larger than unity gain (1.07) with an input of sinusoidal wave with a frequency of 1 GHz ( Fig. 4f ), demonstrating that our amplifier can work in the gigahertz regime with voltage gain, which is advantageous over graphene transistors with which the voltage gain is lacking due to the lack of current saturation. We have performed measurements from 60 MHz to 1.5 GHz and determined the relative voltage gain of our amplifier versus the frequency ( Fig. 4g ). It is clear that our amplifier preserves the relative voltage gain equal to 2 (6 dB) up to 500 MHz, and retains a relative voltage gain >1 at 1 GHz. The propagation delay of MoS 2 amplifier can be probed by applying a square wave generated by an arbitrary waveform generator on the input electrode and measuring the output voltage response by using an oscilloscope. When an input signal with a rise time of 210 ps was applied on the input electrode of our MoS 2 amplifier, an output voltage with a rise time of 580 ps was captured by the oscilloscope ( Fig. 4h ). Considering the delay of input signal, a propagation delay of 370 ps is observed in our MoS 2 amplifier. A square wave is a non-sinusoidal periodic waveform, which can be represented as an infinite summation of sinusoidal waves. By considering the gain for each component of sinusoidal wave, we can simulate the output signal of the propagation delay measurement (detailed calculation in Supplementary Note 1 ). Importantly, the simulated output signal matches well with the experimental results, indicating the proper functionality of our MoS 2 amplifier in the gigahertz regime ( Fig. 4i ). Flexible RF circuits 2DLMs are promising candidates for both flexible and stretchable electronics applications, such as low-power, high-frequency electronics, optoelectronics and integrated systems [48] , [49] . Graphene has been widely speculated for high-performance flexible electronics due to its extremely high carrier mobility and excellent mechanical properties [50] , [51] , but is limited by its semimetal nature and the lack of intrinsic voltage gain. With excellent semiconducting characteristics and few-atomic thickness, MoS 2 is considered an attractive material for high-speed flexible electronics. MoS 2 has been explored for flexible transistors, but typically in d.c. regime to date [11] , [52] , [53] . Importantly, our fabrication approach can be readily applied onto flexible substrate to enable high-performance MoS 2 transistors for low-power flexible electronics ( Fig. 5a ). The self-aligned MoS 2 transistors on flexible substrate (polyimide; see Methods) exhibit a similar performance with a highest current density of 48 μA μm −1 (at V ds =2 V) achieved in a 116 nm channel length MoS 2 transistor on flexible substrate ( Fig. 5b ), greatly exceeding the recent published results [11] . Repeated bending of the MoS 2 transistors (radius of curvature 5 mm) for 1,000 cycles does not apparently affect the performance of the devices ( Supplementary Fig. 9 ). An inverter circuit made from MoS 2 transistors on polyimide substrate exhibits a very sharp transition with a voltage gain ~9 ( Fig. 5c ). 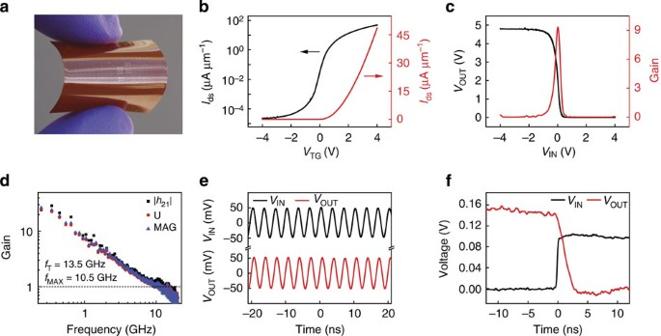Figure 5: Flexible MoS2transistors, integrated logic inverter and RF amplifier. (a) A photograph of MoS2circuits on flexible substrate. (b) TheIds–VTGtransfer characteristics of the device at 2 V bias voltage for the 100 nm channel length top-gated MoS2transistor on flexible substrate. (c) Output voltage (left axis) and the voltage gain (right axis) of the MoS2-based integrated logic inverter as a function of the input voltage under a d.c. bias of 5 V. (d) Small-signal current gain (|h21|), Mason’s unilateral power gain (U) and maximum available gain (MAG) versus frequency for a 68 nm channel length MoS2transistor on flexible substrate at a d.c. bias of 8 V and top-gate bias of 3.7 V. (e) A 300 MHz sinusoidal input signal (black) coupled with 1.2 V d.c. gate bias, and the output signal shows a voltage gain of 1.05. (f) Propagation delay of few-layer MoS2inverter. The input signal (black) has a rise time of 0.2 ns and the output signal (red) has a rise time of 2.2 ns. Figure 5: Flexible MoS 2 transistors, integrated logic inverter and RF amplifier. ( a ) A photograph of MoS 2 circuits on flexible substrate. ( b ) The I ds – V TG transfer characteristics of the device at 2 V bias voltage for the 100 nm channel length top-gated MoS 2 transistor on flexible substrate. ( c ) Output voltage (left axis) and the voltage gain (right axis) of the MoS 2 -based integrated logic inverter as a function of the input voltage under a d.c. bias of 5 V. ( d ) Small-signal current gain (| h 21|), Mason’s unilateral power gain ( U ) and maximum available gain (MAG) versus frequency for a 68 nm channel length MoS 2 transistor on flexible substrate at a d.c. bias of 8 V and top-gate bias of 3.7 V. ( e ) A 300 MHz sinusoidal input signal (black) coupled with 1.2 V d.c. gate bias, and the output signal shows a voltage gain of 1.05. ( f ) Propagation delay of few-layer MoS 2 inverter. The input signal (black) has a rise time of 0.2 ns and the output signal (red) has a rise time of 2.2 ns. Full size image We have further tested the intrinsic RF performance by measuring the intrinsic cut-off frequency ( f T ) and maximum oscillation frequency ( f MAX ) of the MoS 2 FETs on flexible substrate. An intrinsic cut-off frequency ( f T ) of 13.5 GHz and maximum oscillation frequency ( f MAX ) of 10.5 GHz are achieved in a 68 nm MoS 2 FET ( Fig. 5d ), which is lower than those on Si/SiO 2 and quartz ( Supplementary Table 2 ). The lower performance on the plastic substrate may be largely attributed to substrate roughness that could partly degrade the charge transport properties in these atomically thin materials. Moreover, an extrinsic cut-off frequency of 4.7 GHz and a maximum oscillation frequency of 5.4 GHz have been achieved without de-embedding procedures (see Supplementary Fig. 7c ). Taking a step forward, we have also constructed an RF amplifier on flexible substrate based on self-aligned MoS 2 transistors with a channel length of 116 nm and determined its output characteristics. A larger than unity-relative voltage gain was observed in the output signal for a 300 MHz sinusoidal input signal ( Fig. 5e ). Our study represents the first demonstration of MoS 2 circuits on flexible substrate, and as far as we know, there is yet no report of flexible graphene RF circuits with voltage gain above 1 MHz to date. To measure the propagation delay of MoS 2 -based circuits on flexible substrate, a MoS 2 -based inverter was fabricated using two MoS 2 FETs with a channel length of 116 nm. The propagation delay of MoS 2 amplifier on flexible substrate was measured by applying an input signal with a rise time of 0.2 ns on the input electrode of MoS 2 -based inverter ( Fig. 5f , black curve). An inverted output voltage with a rise time of 2.2 ns was captured by the oscilloscope ( Fig. 5f , red curve). Together, a propagation delay of 2 ns is achieved in our MoS 2 amplifier on flexible substrate, demonstrating the potential of MoS 2 transistors for flexible RF applications. In summary, we have demonstrated the best-performed few-layer MoS 2 transistors to date with on–off ratio over 10 7 , intrinsic gain up to 30, intrinsic cut-off frequency up to 42 GHz and maximum power gain performance up to 50 GHz. Importantly, with an intrinsic band gap, the MoS 2 -based transistors can offer several advantages compared with the graphene transistors, including large on/off ratio, excellent current saturation and large intrinsic gain. Exploiting these unique advantages, we have demonstrated that the few-layer MoS 2 transistors can be used to construct functional circuits, including logic inverter and RF amplifier, operating in the gigahertz regime with voltage gain, which is difficult to achieve in graphene-based RF circuit. Our study demonstrates the first MoS 2 -based circuits with current saturation and voltage gain in the gigahertz regime. It represents an important milestone in applying 2DLMs for high-performance electronics, particularly flexible electronics. To properly evaluate the potential of atomically thin MoS 2 for high-speed electronics, it is also useful to compare the RF performance of our MoS 2 transistors with those of graphene and traditional silicon/group III–V semiconductor devices. In general, because of much lower carrier mobility, the highest intrinsic cut-off frequency ( f T ) achieved in MoS 2 (42 GHz) is much lower than that in graphene (up to 427 GHz) [9] . On the other hand, with an intrinsic band gap, the MoS 2 transistors can exhibit much larger on/off ratio, less power consumption and better current saturation behaviour. As a result, the maximum oscillation frequency ( f MAX ) of 50 GHz of the best MoS 2 devices is nearly comparable to that of the best graphene devices ( f MAX =70–105 GHz) [54] , [55] . The achievement of comparable f MAX in MoS 2 with much lower carrier mobility is very notable in the context of 2D electronic materials. Comparing with traditional semiconductors, the RF behaviour of the MoS 2 transistors is only ~1/5th of silicon-on-insulator CMOS technology ( f T =208 GHz and f MAX =243 GHz) with similar gate length (50 nm) [56] , and ~1/10th of typical group III–V devices [43] . At this stage, the MoS 2 transistors cannot compete with traditional silicon or III–V semiconductor technology due to the limitation of the carrier mobility. Nonetheless, considering its much shorter development history than these traditional mature materials, we believe that the performance of MoS 2 or other 2DLM device could be further improved in future studies by reducing the substrate scattering or improving the gate coupling. The atomically thin MoS 2 may represent an interesting alternative for high-speed low-power electronics with excellent potential for the ultimate device scaling due to its atomically thin thickness and superior immunity to short-channel effect [31] . In particular, with the atomically thin carrier transport region and exceptional mechanical strength, these TMD materials may be readily applied onto bendable substrate and are particularly promising for flexible or wearable electronics. It is important to note the maximum oscillation frequency obtained in flexible MoS 2 transistor that here (10.5 GHz) exceeds the best value achieved in graphene flexible transistors ( f MAX ~3.7 GHz) [57] even though a 25 GHz cut-off frequency has been achieved in graphene FET on flexible substrate [51] . The RF performance of our MoS 2 transistors on flexible substrate is also comparable to the best-performed transferred silicon nanomembrane ( f T =3.8 GHz and f MAX =12 GHz) [58] or transferred III–V nanowire FETs ( f T =1 GHz and f MAX =1.8 GHz) [59] on flexible substrate, but is worse than transferred III–V material ( f T =105 GHz and f MAX =22.9 GHz) [60] . On the other hand, with the continued progress in the chemical vapour deposition growth of large-area TMDs, the 2D geometry of the TMD material may also offer better scalability for large-area application than other lower-dimensional materials (for example, nanowires used for flexible electronics) or lower-cost alternative to traditional III–V materials. Device fabrication Few-layer MoS 2 flakes are mechanically exfoliated onto Si/SiO 2 (300 nm), quartz or flexible substrates. The gate stacks—metal bars wrapped in dielectrics—are first patterned on a sacrificial substrate, and then transferred onto the few-layer MoS 2 ( Supplementary Fig. 2 ) using previously reported approach [9] . E-beam lithography (PMMA 495 A4) and vacuum metallization (Ti/Au, 50/50 nm) are then used to define the source, drain and gate electrodes. A thin layer of Ni/Au (5/10 nm) metal is then deposited across the gate stack to form the self-aligned source and drain electrodes. For the MoS 2 devices on flexible substrate, a layer of SU-8 photoresist is spin coated to reduce the surface roughness of flexible substrate before fabricating MoS 2 devices on it. The MoS 2 devices are annealed at 200 °C for 2 h. This annealing step improves the contacts between the self-aligned electrodes and reduces device resistance. Device measurement The d.c. electrical transport measurements are conducted with a Lakeshore vacuum probe station (Model TTP4) and a computer-controlled analogue-to-digital converter (National Instruments model 6030E), DL 1211 current preamplifier and/or Agilent 2902A SMU under vacuum conditions. The on-chip microwave measurements are carried out in the range of 50 MHz–30 GHz using Cascade RF probes and an Agilent 8361A network analyzer under ambient conditions. The measured S parameters are de-embedded using specific ‘short’ and ‘open’ structures with identical layout on the same substrate of the device to remove the parasitic capacitance and resistance associated with the pads and connections. In detail, for ‘open’ structure, the gate stacks are transferred on to desired substrate, followed by E-beam lithography and metallization (Ti/Au, 50/50 nm) process to define the source, drain and gate electrodes. A thin layer of Ni/Au metal with the same area as that of the actual device is then deposited across the gate stack, in which the gate stack separates the Ni/Au thin film into two isolated regions that form the self-aligned source and drain electrodes precisely close to the gate stack. For ‘short’ structure, the stacks are transferred onto desired substrate, followed by the formation of gate and self-aligned source-drain electrodes. Then, the gate stacks and the self-aligned electrodes are shortened by a narrow strip of Ti/Au film. The ‘through’ and ‘load’ calibrations are done with standard calibration pad (Cascade CS-5). The integrated circuit measurements are carried out in Lakeshore probe station (Model TTP4) at room temperature by using an Agilent 81180B arbitrary waveform generator and Fluke 6062A-synthesized RF Signal Generator as the input source, and a Tektronix DPO 5204 oscilloscope (input impedance 1 MΩ) for the output signal detection. SEM and TEM characterization The microstructures and morphologies of the nanostructures are characterized by a JEOL 6700 SEM. The cross-section image of the self-aligned device is obtained by an FEI Titan TEM. How to cite this article: Cheng, R. et al. Few-layer molybdenum disulfide transistors and circuits for high-speed flexible electronics. Nat. Commun. 5:5143 doi: 10.1038/ncomms6143 (2014).